Signature of the Dirac cone in the properties of linear oligoacenes Organic electronics offers prospects of functionality for science, industry and medicine that are new as compared with silicon technology and available at a very low material cost. Among the plethora of organic molecules available for materials design, polymers and oligomers are very promising, for example, because of their mechanical flexibility. They consist of repeated basic units, such as benzene rings, and the number of these units N determines their excitation gap, a property that is often used in proposals of organic photovoltaics. Here, we show that contrary to a widely held belief the magnitudes of excitation gaps do not always decay monotonously with N , but can oscillate due to the presence of a ‘Dirac cone’ in the band structure. With an eye on the more fundamental question how a molecular wire becomes metallic with increasing length, our research suggests that the process can exhibit incommensurate oscillations. Oligoacenes are molecules that consist of fused benzene rings ( Fig. 1a ). The shortest examples—benzene, naphthalene and anthracene—are of fundamental importance in chemistry. While the synthesis of gas-phase oligoacenes with more than six rings (hexacene) remains a challenge [1] , there are reports that attempts are on the way for on-substrate synthesis [2] . On the theory side, oligoacenes have been subject of an intensive debate due to pronounced correlation effects [3] , [4] . Much of the interest in this class of molecules is driven by organic electronics [5] and photovoltaics [6] , [7] , where oligoacenes and their derivatives find frequent applications [8] , [9] , [10] , [11] , [12] . From a broader perspective, a study of systems with linearly fused rings, ‘nano-graphenes’, offers means to learn how properties of a molecular wire converge to the one-dimensional limit. 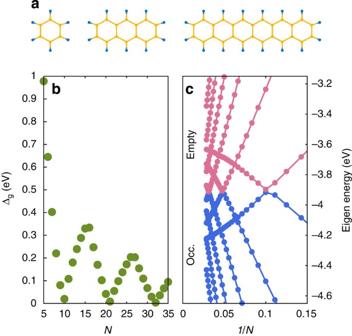Figure 1: Electronic structure of oligoacenes. (a) Ball-and-stick representation of benzene, anthracene and hexacene withN=1, 3, 6 rings (blue: hydrogen, orange: carbon). (b) optical gap of oligoacenes as a function of the number of ringsNcalculated in DFT. (c) Flow of orbital energies as a function of 1/N, showing that a repeating interchange of orbitals occurs as the number of rings grows. Blue symbols are occupied orbitals and red are unoccupied. Close toN=10,N=21 andN=32, there is an interchange of frontier orbitals. The data points are connected by straight lines for visual guidance. Figure 1: Electronic structure of oligoacenes. ( a ) Ball-and-stick representation of benzene, anthracene and hexacene with N =1, 3, 6 rings (blue: hydrogen, orange: carbon). ( b ) optical gap of oligoacenes as a function of the number of rings N calculated in DFT. ( c ) Flow of orbital energies as a function of 1/ N , showing that a repeating interchange of orbitals occurs as the number of rings grows. Blue symbols are occupied orbitals and red are unoccupied. Close to N =10, N =21 and N =32, there is an interchange of frontier orbitals. The data points are connected by straight lines for visual guidance. Full size image As the number of fused molecular units increases, the optical gap either approaches a constant or vanishes. In the former case, the infinite chain is a band insulator and in the latter it is a metal. Metallic behaviour is usually manifested by a single band that crosses the Fermi energy. This band is partially filled and the gaps of chains of finite length should tend to zero as quickly as 1/ N , N being the number of units. The 1/ N behaviour merely reflects the well-known level spacing of the particle-inside-a-box model. Hence, the common belief that the decay is generally monotonous (possibly, with decorating even-odd oscillations). However, in this work, we demonstrate that the gap can decay in a non-monotonous way, with strong and even incommensurate oscillations. Our calculations based on density-functional theory (DFT, detailed in Methods) show that the gap of the first 10 oligoacenes drops to zero quickly, but it rises up again and drops repeatedly with periodicity of 11 units (rings). By a sophisticated post-DFT analysis, we clarify the conditions for observing the oscillations in oligoacenes. Remarkably, this behaviour has not been reported before in spite of the intensive research focus on these molecules. As we argue below, the gap oscillations originate from a band crossing at the Fermi level, that is reminiscent of the Dirac points and Dirac cones in certain films, such as graphene, and bulk materials. A consequence of the oscillations is that molecules with similar excitation gaps can have very different lengths. In practical terms, our research implies that the molecular length can be a parameter that can be optimized in addition to the energy gap. Single-particle spectrum The segmented (piecewise-smooth) form of the oligoacene gap, shown in Fig. 1b , indicates that an orbital crossing occurs at the extremal points of the gap function. We confirm this by inspecting the Kohn–Sham eigenvalue spectra in Fig. 1c . The orbital energies evolve as almost straight lines as a function of the inverse chain length and create a web-like pattern. For a given N , the highest occupied molecular orbital (HOMO) is given by the blue symbol of the highest energy; the lowest unoccupied molecular orbital (LUMO) corresponds to the red symbol of the lowest energy. Close to certain crossings, the LUMO and HOMO interchange—in this situation, the gap has a minimum. The local maxima of the gap manifest another level crossing. Band crossing To understand the origin of the oscillations and level crossings, we invoke the band structure of the infinite chain, ‘polyacene’, in Fig. 2 . As one passes from the Γ point towards the corner of the Brillouin zone, we encounter a crossing of the valence and conduction bands at k D =0.9102 π / a . This peculiar band structure of polyacene wires was discussed first by Kivelson and Chapman [13] based on an analysis of a tight-binding Hamiltonian with first ( t ), second ( t ′) and third nearest neighbour hopping ( t ′′). As they argued, t ′′ shifts the conduction and valence bands against each other. If t and t ′′ share the same sign, the shift is negative and we witness a non-avoided band crossing. From our DFT-calculation, Fig. 2 , we estimate t ′′=0.1 t =0.31 eV by matching to the tight-binding model. 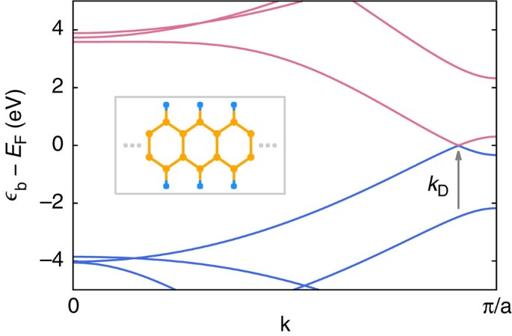Figure 2: Band structure of polyacene highlighting the band crossing at a Dirac point. Blue lines are occupied bands, red lines are unoccupied. The gap between the valence and conductance bands decreases as we move from the Γ point (k=0) to the zone border, where it becomes negative.a=2.462 Å is the unit cell length. The band structure was calculated in DFT, see Methods for details. Inset: ball-and-stick model of polyacene with carbon (yellow) and hydrogen (blue) atoms. Figure 2: Band structure of polyacene highlighting the band crossing at a Dirac point. Blue lines are occupied bands, red lines are unoccupied. The gap between the valence and conductance bands decreases as we move from the Γ point ( k =0) to the zone border, where it becomes negative. a =2.462 Å is the unit cell length. The band structure was calculated in DFT, see Methods for details. Inset: ball-and-stick model of polyacene with carbon (yellow) and hydrogen (blue) atoms. Full size image As a consequence of crossing, electrons and holes with energies sufficiently close to the Fermi level have a piecewise linear dispersion (see Fig. 2 ) reminiscent of the Dirac cones in graphene. Just as in graphene, the ‘Dirac point’ in polyacene is a property of the conjugated π electron system. However, in graphene, the position of the Dirac points in the Brillouin zone is dictated by the symmetry of the honeycomb lattice, while in polyacene it is controlled by t ′′. Origin of oscillations At least in the case of sufficiently long oligoacenes, one should be able to derive their spectrum from the polyacene band structure by imposing selection rules for wave numbers due to hard-wall boundary conditions (‘zone-folding’). For a given number of rings N , only selected wave numbers are allowed. We choose the following set which applies for a guitar string of the length a ( N +1), a is the length of one ring. In Supplementary Note 1 , we inspect the boundary condition in detail and demonstrate in Supplementary Fig. 2 that the optimal quantization length is the one given in equation 1. Let us denote E g ( k ) := ε c ( k )− ε v ( k ), where ε c,v are the conduction and valence band energies. The optical gap will be given approximately by the energy , where denotes the wave number from the allowed set, that is closest to the Dirac point, k D . Hence, labels the HOMO/LUMO pair. As we increase the number of rings, will move and eventually cross the Dirac point, where the HOMO and LUMO interchange. This explains that the periodicity of the gap oscillations of the oligoacenes is controlled by the position of the Dirac cone in the Brillouin zone. More precisely, the period is inversely proportional to π / a − k D , the distance to the zone boundary. Similarly, the maxima of the gap are also fixed by band structure consideration: it is only when the Dirac point lies in the middle between two consecutive wave numbers from the allowed set. If a local maximum occurs at N 0 with value , its upper bound must be ℏ υ F π / a /( N 0 +1), where υ F is the Fermi velocity (numerically ℏ υ F π / a =6.485 eV). The above considerations suggest natural energy and length scales. In Fig. 3 , we show the gap expressed in these natural units (blue trace). Remarkably, our plotting exhibits a sawtooth form with well developed periodicity (with the exception of very small molecules). Furthermore, in the same plot we show —the gaps reconstructed from folding the polyacene band structure (red traces). Remarkably, both traces lie almost on top of each other. Naively, corrections of the order of 1/ N to the zone-folding procedure should be expected, which means a correction of the order of 100% for benzene, N =1. In practice, the finite-size correction turns out to be much smaller. For benzene, the deviation is only 11% (tetracene 1%, hexacene 8%). We comment that the molecular gaps in Fig. 3 already involve relaxation effects that can not be accounted for in the zone folding. We see that is always higher than for N >4. We attribute this to the fact that the relaxation effects compress the length of the rings at molecule’s edges. Since the total length shrinks, the level spacing and gap increase. 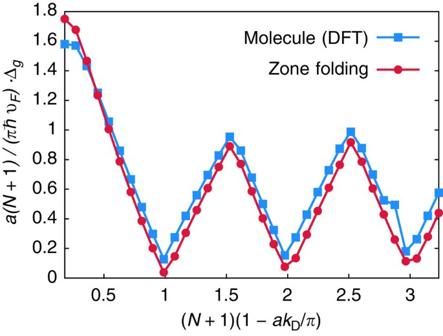Figure 3: Comparison of optical gaps of oligoacenes from DFT and zone folding. The gap energies are divided by the factorπℏυF/(N+1)/ato scale away the leading behaviour. The horizontal axis is rescaled by the reciprocal space distance of the Dirac point to the zone border. Blue squares are calculated for a set of geometry-optimized molecules from DFT. Red circles are calculated from the Bloch bands of the infinite chain by Brillouin zone folding. The data points are connected by lines for visual guidance only. Figure 3: Comparison of optical gaps of oligoacenes from DFT and zone folding. The gap energies are divided by the factor π ℏ υ F /( N +1)/ a to scale away the leading behaviour. The horizontal axis is rescaled by the reciprocal space distance of the Dirac point to the zone border. Blue squares are calculated for a set of geometry-optimized molecules from DFT. Red circles are calculated from the Bloch bands of the infinite chain by Brillouin zone folding. The data points are connected by lines for visual guidance only. Full size image We have seen that on DFT level, band structure effects control the excitation gaps of oligoacenes. It is known that the Kohn–Sham excitation gaps obtained from the DFT ground-state calculation agree with optical excitations only up to corrections that are incorporated in time-dependent DFT. These corrections include a Hartree and an exchange-correlation kernel that can renormalize the excitation energies. In ref. 14 , these dynamical correction have been calculated for the smaller system sizes N =2–6 (with a hybrid functional) and turn out to be below 10% of the bare Kohn–Sham gap. As screening effects generally enhance with decreasing gap, that is, increasing system size, it is reasonable to expect that dynamical corrections do not affect the picture that we present. Charged excitations We now argue that the charged excitation energies, that is, the ionization energies and electron affinities, also inherit the oscillatory structure from the ‘Dirac cone’. In this section, we provide an analysis of results by DFT and various post-DFT techniques. The latter can exhibit significant deviations from the DFT estimates and therefore correct for artifacts of approximate exchange-correlation functionals [14] , [15] , [16] . As it is well known, in KS–DFT, the ionization potential I agrees with the HOMO energy of the charge-neutral molecule with N el electrons: I =− ε HOMO ( N el ). The corresponding electron affinity A can be obtained from a reference calculation that has been performed with one additional electron: A =− ε HOMO ( N el +1). In contrast to DFT, in Green's function methods (such as G 0 W 0 ), the energies of charged excitations are already incorporated in the quasiparticle (QP) energies. The G 0 W 0 QP band structure is shown in Supplementary Fig. 1 . It shows a band pattern very similar to the DFT results. Since computational demands do not allow a fine resolution near the Fermi points, we inspect the symmetry of the four Bloch states in Fig. 4 , which provides evidence of a band crossing in G 0 W 0 . Therefore, one expects that the charged excitations support oscillations analogous to the ones already observed in the optical gaps. The renormalized parameters of the Dirac cone are compared in Supplementary Table 1 . 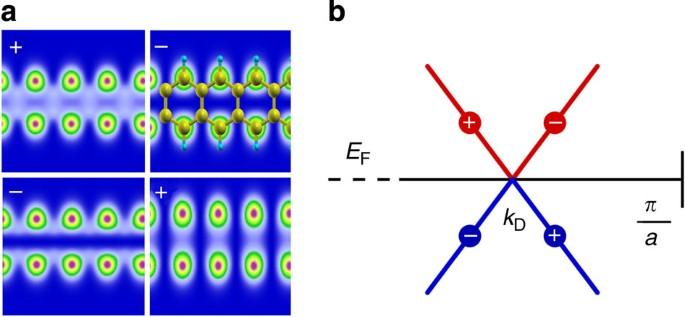Figure 4: Evidence of band crossing inG0W0. (a) Charge density of QP states of polyacene in theG0W0approximation. We plot charge density in the plane offset by 0.7 Å from the molecular plane. The colour changes linearly from blue, corresponding to zero. Shown are four states whose energies lie in the vicinity of the Fermi level, as sketched inbby four circles. The QP band whose energy grows withkhas a nodal plane along the C–C bonds of the rungs and we indicate it by the − sign. The other two states that pertain to the band of decreasing energy are labelled as + and lack the nodal plane. Figure 4: Evidence of band crossing in G 0 W 0 . ( a ) Charge density of QP states of polyacene in the G 0 W 0 approximation. We plot charge density in the plane offset by 0.7 Å from the molecular plane. The colour changes linearly from blue, corresponding to zero. Shown are four states whose energies lie in the vicinity of the Fermi level, as sketched in b by four circles. The QP band whose energy grows with k has a nodal plane along the C–C bonds of the rungs and we indicate it by the − sign. The other two states that pertain to the band of decreasing energy are labelled as + and lack the nodal plane. Full size image In what follows, we will represent the number of rings N by a dimensionless number ξ =( N +1)(1− ak D / π ), where k D is the Dirac wave number and a is the lattice parameter. Brillouin zone folding predicts gap minima at integer ξ . The orbital energies E i ( i stands for HOMO or LUMO) will be represented by a dimensionless quantity . First, we discuss the behaviour of the HOMO and LUMO (Kohn–Sham) energies on DFT–Perdew–Burke–Ernzerhof (PBE) level. The LUMO energy enters because we replace ε HOMO ( N el +1) by ε LUMO ( N el ) thus ignoring effects of the derivative discontinuity. In Fig. 5 , we show HOMO (symbols red, filled) and LUMO energies (symbols red, open), along with their counterparts from the Brillouin zone folding (solid lines). As expected, with increasing number of rings the frontier orbitals cross near ξ =1 in a linear fashion. 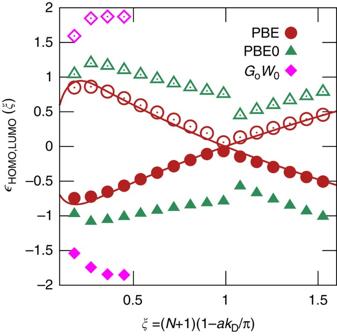Figure 5: Comparison of charged excitation energies obtained with different methods. We plot dimensionless HOMO and LUMO energies, over the length of the oligoacene. The parametersa,υF,EFandkDwere obtained from a separate PBE band structure calculation. PBE results are represented by red symbols; red lines are estimates from Brillouin zone folding. Green symbols represent the PBE0 counterparts and magenta are theG0W0QP energies. Empty (filled) symbols stand for LUMO (HOMO). Figure 5: Comparison of charged excitation energies obtained with different methods. We plot dimensionless HOMO and LUMO energies , over the length of the oligoacene. The parameters a , υ F , E F and k D were obtained from a separate PBE band structure calculation. PBE results are represented by red symbols; red lines are estimates from Brillouin zone folding. Green symbols represent the PBE0 counterparts and magenta are the G 0 W 0 QP energies. Empty (filled) symbols stand for LUMO (HOMO). Full size image The frontier orbitals can be classified according to the symmetry with respect to a mirror plane that is normal to the molecular plane cutting the molecule along the long axis into two identical pieces. Notably, the energy of symmetric (antisymmetric) orbitals decreases (increases) with ξ . Hence, at ξ =1, the band theory predicts a change in the symmetry of the HOMO orbital. The reverse symmetry transitions appear at half-integer steps in ξ . We have verified that this is indeed the case for the molecules calculated in PBE. In the following, we explore an interesting consequence of the symmetry transition for the energies of charged excitations. To this end, we present HOMO and LUMO energies calculated in PBE0. PBE0 is a (hybrid) density functional that replaces a certain fraction λ of the PBE exchange by an exact (Hartree–Fock type) exchange. In conventional PBE0, one takes λ =25%. The derivative discontinuity, that is absent in PBE, is thus partially restored. In Fig. 5 , the (dimensionless) PBE0 energies ε HOMO,LUMO are shown (green symbols). They deviate significantly from the PBE zone-folding estimates. This difference is due to λ : it vanishes continuously in the limit λ →0. The PBE0 data brings two qualitatively new features. With hybrid functionals, LUMO and HOMO energies contain a fraction of the charging energy. In PBE0, the latter is entirely given by Hartree–Fock exchange, which does not account for interaction screening. Hence, for long linear chains, the charging energy will be dominated by a spurious logarithmic length dependence. The slowly increasing deviation between the HOMO/LUMO energies and band lines for the first 10 molecules can be understood in this way. At N =11, we witness an abrupt change: a slope inversion and a step in the PBE0 trace. It can be understood in the following way. The electronic structure data for PBE0 and PBE are adiabatically connected via the λ parameter. Hence, for every system size N , the frontier energies obtained with PBE0 can be thought of as originating from a PBE reference result corrected by perturbative terms that are controlled by λ . The correction terms describe the charging energy and therefore contain Coulomb-matrix elements of the PBE reference calculation. At N =11, the symmetry of the frontier orbitals of the PBE reference calculation changes. The Coulomb-matrix elements react to that change and consequently the PBE0 traces exhibit a jump. In the presence of screening beyond PBE0, we expect that the spurious logarithm disappears in the limit ξ →∞ and the step will be weaker. The G 0 W 0 QP energies are also shown in Fig. 5 . It is easy to understand the differences between all methods presented if we recall that the PBE0 values contain a fraction of the charging energy, while the G 0 W 0 values fully include charging effects. Consequently, for benzene, the difference in orbital energies is approximately four times the difference and the same holds true for LUMO. We notice that for longer molecules, the relative difference drops below four, because of the screening mechanism in G 0 W 0 that is absent in PBE0. Due to high computational demands, we could not obtain QP energies for systems beyond N >4 rings. Correlation effects To rigorously establish the validity or our conclusions even in the presence of strong correlations (where ab initio methods tend to fail), we analyse a (parameterized) model system, the oligoacene Hubbard model. We solve it numerically at different values of the interaction strength by employing the density-matrix renormalization group (DMRG), see Methods for details. We first discuss a model with spin-less fermions. Results for the optical gap are show in Fig. 6 for various values of N and nearest neighbour interaction U 1 . As we see, the N oscillations of the optical gap survive even up to interactions comparable in strength with the bandwidth. The period can be renormalized to the extent that for large interaction the oscillation period increases. At a certain critical value comparable to the bandwidth, U 1 ≈5 eV, the period diverges. At large interactions U 1 >>5 eV, we find a (twofold degenerate) nearest neighbour charge density wave ground state. 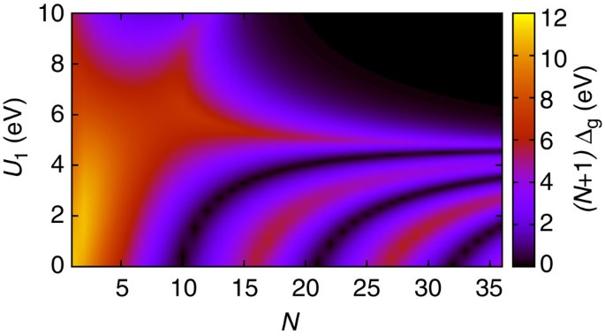Figure 6: DMRG results of the optical gap in the spin-less case with varying interaction strength. With growing interactions the oscillation period increases until it diverges at an interaction strength approximately equal to the bandwidth. Figure 6: DMRG results of the optical gap in the spin-less case with varying interaction strength. With growing interactions the oscillation period increases until it diverges at an interaction strength approximately equal to the bandwidth. Full size image Our DMRG results for the spin-full calculation at low interaction strength are depicted in Fig. 7a . The data confirms that the oscillation phenomenon is stable against the presence of weak interactions. 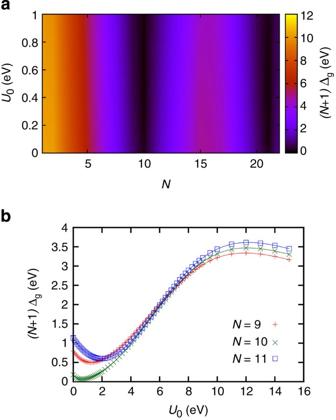Figure 7: DMRG results of the optical gap for a spin-full Hubbard model. (a) Oscillations in the optical gaps are stable for small interactionsU0(vertical scale). The interaction has little or no influence on the period of the oscillations. (b) gaps for increasing on-site interactionU0for system sizesN=9,10 and 11, which are close to the first minimum of the optical gap. (Lines are guides to the eye.). Figure 7b displays the dependency of the optical gap on the on-site interaction, U 0 . Three molecules are shown with a length N that is close to the optimal length N min ≈10 where the gap is expected to exhibit particularly small excitation gap. In the perturbative regime U 0 ≪ 2 t , switching on U 0 even stabilizes the oscillations and makes them more pronounced in the sense that the ratio between the minimal gap near N min ≈10 and the neighbouring gaps goes through a maximum at finite U 0 . At interaction strength U 0 ≲ 2 t , the excitation energy for N =10 is significantly smaller than for the neighbouring molecules N =9,11. Only at U 0 ≈6 eV, the two traces ( N =9,10) cross. At larger values, a monotonous order (in N ) of the traces is established. Figure 7: DMRG results of the optical gap for a spin-full Hubbard model. ( a ) Oscillations in the optical gaps are stable for small interactions U 0 (vertical scale). The interaction has little or no influence on the period of the oscillations. ( b ) gaps for increasing on-site interaction U 0 for system sizes N =9,10 and 11, which are close to the first minimum of the optical gap. (Lines are guides to the eye.). Full size image By performing an independent DMRG calculation in the spin-sector S =1, we have checked that the optical gap coincides with the spin gap for the values of U considered in this manuscript. The scaling of the excitation gap with system size is shown in Fig. 8 . 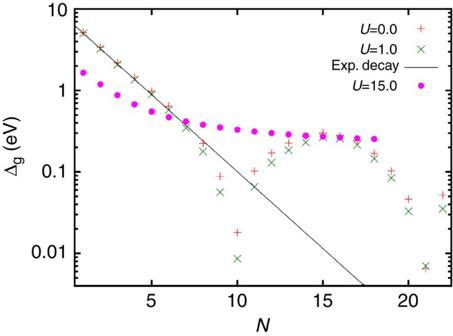Figure 8: Scaling the optical gap with the number of ringsNin the spin-full model. Traces with three values of the on-site Hubbard interactionU0=0,1.0,15.0 eV are shown. For smaller molecules, an approximately exponential decay is observed that can be fitted by Figure 8: Scaling the optical gap with the number of rings N in the spin-full model. Traces with three values of the on-site Hubbard interaction U 0 =0,1.0,15.0 eV are shown. Full size image with Δ 0 ≈7.8 eV and N *≈2.3. Since the quasiexponential decay is already seen at weak interactions including U 0 =0, it is unrelated to correlation effects, such as ground state magnetism. Interaction effects become relevant only at N ≳ N * and very strong values of U 0 that significantly exceed the bandwidth ≈2 t . In this regime, the gap oscillations disappear and a monotonous behaviour sets in, see Fig. 8 Over the years, there has been intensive theoretical and experimental work that addresses the nature of the ground-state of oligoacenes, for review, see refs 1 , 4 . The topic of interest is whether the ground state could be magnetic (open shell, radical) or at least close to a magnetic (or other) instability. We discuss a selection of earlier work that appears most relevant to us in the light of our new findings. In DFT studies employing hybrid functionals, broken-symmetry, spin-polarized ground states have been reported [17] . Since approximate functionals underestimate quantum fluctuations, they tend to overestimate the tendency for symmetry breaking. Therefore, such studies are difficult to interpret. Indeed, our DMRG calculations indicate that the ground state does not exhibit a (simple) broken-symmetry phase. To be consistent with this finding, we employ in our DFT studies non-magnetic, closed-shell calculations. To address correlation effects, other methods have been applied. Where only relatively small system sizes could be addressed, an extrapolation of excitation energies to the polymer-limit of large N was performed (theory [3] N ≤12, experiment [18] N ≤6). For instance, Hachmann, et al. [3] performed a DMRG study on a model of polyacene similar to ours. These authors fit their data for the spin-triplet gap in the manner Δ E st ≈Δ st + δ st exp(− N / N st ) with a non-vanishing offset Δ st ≈0.144±0.017 eV (orig: 3.33±0.39 kcal mol −1 ). The offset indicates the presence of strong correlations that have been interpreted as a singlet ground state with an open shell (di- or polyradical). A finite offset has also been reported in another DMRG study on an oligoacene-like Heisenberg model (up to N =28) [19] . Since the Heisenberg Hamiltonian ignores charge fluctuations, the latter result carries over to oligoacenes only in the Mott-limit of very large U 0 . In this regime, our results are consistent with refs 3 , 19 in the sense that we confirm the absence of oscillatory behaviour, as shown in Fig. 8 for very large interaction U ≳ 2 t . In this regime, our results are also in agreement with the study of ref. 20 where in the large U limit an enhanced ‘mottness’ for an honeycomb like two-leg ladder in comparison to a quadratic two-leg ladder was shown. In conclusion, we show by a combination of DFT, post-DFT methods ( GW theory) and numerically exact Hubbard-type model calculations that oligoacenes exhibit oscillations in their fundamental excitation gaps with increasing length N . It has been shown that these oscillations result from the well-known ‘Dirac-type’ dispersion of polyacene in combination with a zone-folding argument. This basic origin suggests that the effect is robust, which is an important requirement for prospective technological applications. We have seen that the oscillatory modulation of the gap dependence may be hindered if strong interactions are active. At present, a realistic estimate of the interaction strength is lacking. However, even if the Coulomb repulsion wipes out gap oscillations in the gas phase, our study suggests that these band structure effects will revive when molecules are embedded in screening environments, such as electrochemical solutions [21] or synthesized on surfaces, where the effective screened interaction will be several times reduced as compared with the gas-phase value. Density-functional calculations We employ the usual Kohn–Sham density-functional method [22] , [23] implemented in the Fhi-Aims package [24] . The optical gaps were calculated using the Perdew–Burke–Ernzernhof [25] functional. The spin-restricted (closed shell) Kohn–Sham equations were solved in a non-relativistic form, with relativity included a posteriori by rescaling the Hamiltonian eigenlevels, according to the zeroth order regular approximation [26] . The basis set for hydrogen (carbon) contained totally 15 (39) functions of angular momenta up to l =4 and distinct radial dependences (the basis set is called tier2). For periodic calculation of the band structure, we sampled the Brillouin zone using 1,000 points in the reciprocal chain direction. For both periodic and non-periodic calculations, the ground state was reached with strict convergence criteria for the difference in density (10 −6 ), total energy (10 −7 eV) and forces (10 −5 eV Å −1 ). Geometries were considered optimized only after the maximum residual force dropped bellow 10 −3 eV Å −1 . The optical gap, shown in Figs 1 and 2 , was approximated as the energy difference between the LUMO and the HOMO. A discussion of effects beyond this approximation is included in Results. The G 0 W 0 calculations For the QP band structure and QP spectra of finite chains, we have used Vienna Ab initio Simulation Package (VASP) [27] , [28] . In VASP, the one-electron orbitals are expressed using the projector augmented wave basis set [29] . In this calculation, we used plane waves with 400 eV energy cutoff for the DFT starting calculation, and a cutoff of 300 eV for the response functions. First, standard Kohn–Sham DFT calculations were performed, using the PBE [25] exchange-correlation functional. Then, QP corrections were included on top of the Kohn–Sham states at the non-self-consistent, single-shot, G 0 W 0 level. After convergence checks, a frequency grid of 80 points and 600 bands in total was used. The QP energies were represented on a mesh of 11 k -points in the Brillouin zone. The oligoacene Hubbard model and DMRG Following Kivelson and Chapman [13] , we construct a tight-binding model with a single orbital site per carbon atom at half filling and including up to third nearest neighbour hoppings t , t ′ and t ′′. We set t =3.1 eV, t ′=0.341 eV, t ′′=0.31 eV (as estimated from our ab initio band structure). We allow for on-site ( U 0 ) and nearest neighbour ( U 1 ) interactions, that we take as a variable parameters. We perform an analysis based on the DMRG. DMRG is a well-established method suitable for studying many-body eigenvalue spectra of quasi-one-dimensional systems with strong correlations [30] , [31] . We study the oligoacene Hubbard model in a spin-less and spin-full fashion. In the spin-less case, we take U 1 variable ( U 0 is meaningless). Discarded entropies during the DMRG sweeps are always below 10 −7 , typically much lower. In the spin-full case, results are parameterized by U 0 , while U 1 =0. We keep up to 8,000 states per block; the dimension of the target space grows up to 4.3 × 10 7 , the discarded entropies are considerably below 10 −4 (even for N =21) in each DMRG step, typically significantly smaller. We employ at least seven finite lattice sweeps with an optimized infinite lattice warm up. The optical gap is the difference between first excited and ground-state energies. How to cite this article : Korytár, R. et al. Signature of the Dirac cone in the properties of linear oligoacenes. Nat. Commun. 5:5000 doi: 10.1038/ncomms6000 (2014).